Image-guided radiotherapy platform using single nodule conditional lung cancer mouse models Close resemblance of murine and human trials is essential to achieve the best predictive value of animal-based translational cancer research. Kras -driven genetically engineered mouse models of non-small-cell lung cancer faithfully predict the response of human lung cancers to systemic chemotherapy. Owing to development of multifocal disease, however, these models have not been usable in studies of outcomes following focal radiotherapy (RT). We report the development of a preclinical platform to deliver state-of-the-art image-guided RT in these models. Presence of a single tumour as usually diagnosed in patients is modelled by confined injection of adenoviral Cre recombinase. Furthermore, three-dimensional conformal planning and state-of-the-art image-guided dose delivery are performed as in humans. We evaluate treatment efficacies of two different radiation regimens and find that Kras -driven tumours can temporarily be stabilized upon RT, whereas additional loss of either Lkb1 or p53 renders these lesions less responsive to RT. Despite recent advances in therapeutic options, lung cancer remains the leading cause of cancer-related deaths in the United States [1] . In particular, improved radiation treatment modalities like stereotactic body radiation therapy (SBRT) have led to 3-year local control rates of around 90% in Stage I non-small-cell lung carcinomas (NSCLCs) [2] , [3] . The concept of SBRT comprises delivery of very high doses of ionizing radiation (IR) given in a single or small number of fractions to the tumour volume, while minimizing the radiation exposure of non-targeted tissue. However, recent knowledge about molecular alterations leading to activation of a multitude of oncogenic drivers in NSCLC is currently not applicable to RT stratification because we still lack sound understanding of how these mutations mechanistically affect the radiation sensitivity within a given tumour. Upon our recent observation that additional alterations in Kras -driven murine NSCLC have distinct impacts on therapeutic response to systemic chemotherapy [4] , we suspect that similar genotype-dependent differences may affect RT sensitivity. Taking into consideration the multiplicity of identified genomic alterations in NSCLC and potential treatment regimens, the utilization of predictive preclinical models appears to be a valid tool to preselect the most promising treatment regimens before more costly and time-consuming clinical studies. Despite a large body of literature describing in vivo RT studies, the majority of these experiments were performed in conventional xenograft models. Among the associated limitations with these models are: ectopic implantation of cancerous cells, lack of a functional immune system and altered tumour vasculature. Two recent studies report on model improvements by orthotopic transplantation of human lung cancer cells for studying radiation biology in vivo [5] , [6] . A valid approach to overcome these shortcomings uses genetically engineered mouse models (GEMMs). Tumours of these models closely recapitulate the genetic and histopathological features of human disease [7] . GEMMs not only allow for autochthonous tumour formation surrounded by a normal tissue microenvironment in an immunocompetent animal, but also offer the possibility to model any gene mutation that is relevant in human lung cancer. Two studies of RT response in lung cancer GEMMs have been published recently, but these mice did not have isolated tumour nodules to allow for precise focal RT [8] , [9] . Thus, the systematic preclinical study of RT efficacy in genetically distinct subtypes of NSCLC ideally meets the following criteria to predict therapeutic response in humans as closely as possible: (i) employment of lung cancer-relevant GEMMs; (ii) application of target delineation and treatment delivery as performed in humans and (iii) utilization of treatment regimens currently employed in humans. In the present work, we report the development of a preclinical platform, which encompasses all of the outlined requirements above: 1 We utilize three distinct GEMMs of primary lung adenocarcinoma. Upon application of Cre, oncogenic Kras G12D is activated [10] , and deletion of a tumour-suppressor gene, either Lkb1 (also known as Stk11 ) [11] or p53 (also known as Tp53 ) [12] is initiated. 2 We establish a new technique, which allows for single lung tumour nodule formation by directly introducing Cre recombinase into a small number of lung epithelial cells. We perform three-dimensional conformal radiotherapy planning (3DCRT) and state-of-the-art image-guided RT (IGRT) delivery as performed in humans. 3 We compare treatment efficacy of two RT regimens—five fractions of 4 Gy and two fractions of 8.5 Gy representing two commonly employed hypofractionated RT regimens that are used in patients [13] , [14] —in Kras G12D (K) mice and find that these tumours can temporarily be stabilized upon RT. Furthermore, we evaluate therapeutic efficacy of RT in Kras G12D ;Lkb1 L/L (KL) and Kras G12D ;p53 L/L (KP) mice and observe that these lesions are less responsive to RT in comparison to K tumours. Development of Cre-controlled single focus murine NSCLC In humans, lung cancer is thought to arise from a few cells that carry a series of somatic mutations causing activation of oncogenes and/or inactivation of tumour suppressors [15] . To recapitulate this tumour-initiation step, we performed region-specific injection of adenoviral Cre recombinase into the left lung lobe to establish a solitary tumour nodule ( Fig. 1 ). In comparison, NSCLC formation in these GEMMs is commonly initiated by either intranasal or intratracheal application of Adeno-Cre (AdCre), which leads to multifocal disease in all five lung lobes ( Fig. 1a , left panel) [16] . Importantly, our novel approach of intrathoracic application of AdCre was found sufficient to yield solitary KL tumour nodules of 50–175 mm 3 within 3–4 weeks ( Fig. 1b and Supplementary Fig. 1 ). However, as tumour latency varies among mice of the same genotype, either clinical or non-invasive imaging methods are necessary to screen for tumour-bearing mice. 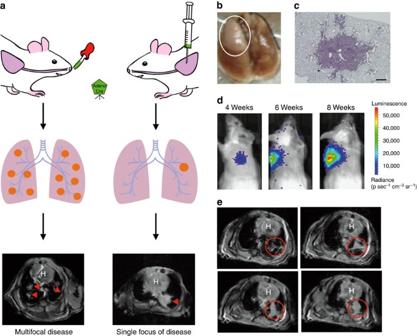Figure 1: Induction of solitary murine lung cancer tumours. (a) Schematic comparison of Cre recombinase-dependent induction methods in conditional mouse lung cancer models. Left panel: intranasal or intratracheal Adeno-Cre application results in multifocal disease as visualized by MRI (arrow heads). Right panel: intrathoracic Adeno-Cre application yields a single focus of disease in the left lung lobe (arrow head). (b) Macroscopic dorsal view on dissected tumour-bearing murine lungs from aKLmouse at 4 weeks post AdCre induction. (c) Haematoxylin and eosin-stained lung tumour from aKmouse at 9 weeks post AdCre administration. Scale bar, 500 μm. (d) Tumour progression ofKLPmurine lung tumour induced with Lenti-Luc.Cre measured by bioluminescence at the indicated time points either in left lateral or dorsal view. (e) Corresponding MRI scan (axial view) ofKLPmouse fromdat 8 weeks post Lenti-Luc.Cre application. Tumour circled in red. H, heart. Hence, we considered non-invasive bioluminescence imaging as a valid alternative to screen for tumours ( Fig 1d,e ). To assess this approach, we injected lentiviral particles encoding Luciferase and Cre recombinase (Lenti-Luc.Cre) into Kras G12D ;Lkb1 L/L ;p53 L/L ( KLP) mice and followed tumour progression in the left lung over 4 weeks starting 4 weeks post-infection ( Fig. 1d ). We performed magnetic resonance imaging (MRI) on the same animal 8 weeks after tumour induction to establish correlation between bioluminescence signal and tumour volume ( Fig. 1e ). Figure 1: Induction of solitary murine lung cancer tumours. ( a ) Schematic comparison of Cre recombinase-dependent induction methods in conditional mouse lung cancer models. Left panel: intranasal or intratracheal Adeno-Cre application results in multifocal disease as visualized by MRI (arrow heads). Right panel: intrathoracic Adeno-Cre application yields a single focus of disease in the left lung lobe (arrow head). ( b ) Macroscopic dorsal view on dissected tumour-bearing murine lungs from a KL mouse at 4 weeks post AdCre induction. ( c ) Haematoxylin and eosin-stained lung tumour from a K mouse at 9 weeks post AdCre administration. Scale bar, 500 μm. ( d ) Tumour progression of KLP murine lung tumour induced with Lenti-Luc.Cre measured by bioluminescence at the indicated time points either in left lateral or dorsal view. ( e ) Corresponding MRI scan (axial view) of KLP mouse from d at 8 weeks post Lenti-Luc.Cre application. Tumour circled in red. H, heart. Full size image Dose planning and state-of-the-art image-guided irradiation One of the known toxicities of thoracic radiation treatments involves radiation dose to the surrounding normal lung tissue. To minimize collateral damage, 3DCRT with multiple highly conformal beams is used in humans. Although two recent studies—also employing GEMMs of NSCLC in RT experiments—do not report any severe acute toxicities after whole lung RT with 15.5 and 14.6 Gy, respectively [8] , [9] , this does not accurately model the therapeutic situation in human patients. Increasing evidence of promising combinatorial treatment regimens of RT and immunomodulatory agents strongly argues for precisely targeted RT to avoid the impact of RT-induced lymphocyte killing or the exacerbation of out-of-field inflammation [17] , [18] . In the present work, we describe for the first time, 3DCRT planning in a preclinical model of NSCLC ( Fig. 2 ). After acquisition of a pre-treatment MRI scan in a manner similar to a patient receiving diagnostic axial imaging ( Fig. 2a ), mice were subjected to cone beam computed tomography (CBCT) in the prone position to enable real-time image guidance for target delineation ( Fig. 2b ). 3DCRT planning of the prescribed dose was done on axial planes of the radiation planning scan ( Fig. 2c–e ). Close resemblance to RT delivery in humans was achieved by using two conformal beams per fraction. The lateral beam ( Fig. 2c , red line) was applied to the left chest at an angle of 90° to the treatment table. The dorsal beam ( Fig. 2c , white line) was applied to the back in an angle of 10° to avoid direct irradiation of the spinal cord. In the present simulation, the isocentre (IsoC) was placed in the middle of the tumour and a 5 × 5 mm 2 collimator was used to encompass the tumour volume ( Fig. 2d , blue lines). The collimator size for treatment was chosen based on coverage of the imaged tumour. Finally, the radiation dose distribution around the volume to be treated was visualized using a dose wash. The prescribed dose was 8.5 Gy in one fraction ( Fig. 2e,f ). The rapid fall-off of the radiation dose beyond the prescribed isodose is clearly seen by minimal colouring of the surrounding tissues. 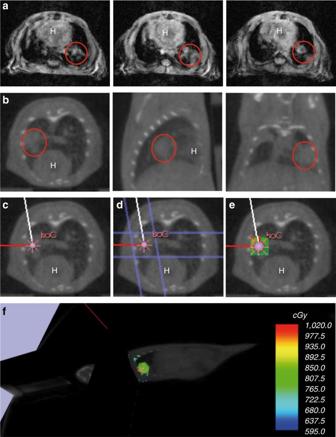Figure 2: Image-guided small animal dose planning system for precise targeted irradiation. (a) MRI scan of aKLmouse at 3 weeks post AdCre application, axial view. Tumour circled in red. (b) Corresponding CBCT scan of aKLmouse, (a) axial view (left panel), sagittal view (middle panel) and coronal view (right panel). Tumour circled in red. (c) Simulation of beam angles: red line represents 90° left lateral beam, white line represents 10° left dorsal beam. (d) Simulation of both involved fields (flanking blue lines) using a 5 × 5 mm2collimator. (e) Simulation of radiation dose distribution around the treatment volume. The prescribed dose was 8.5 Gy in one fraction. (f) Sagittal view ofe(mouse head on the left). Rapid fall-off of the radiation dose beyond the prescribed isodose is visualized by colour wash. Figure 2: Image-guided small animal dose planning system for precise targeted irradiation. ( a ) MRI scan of a KL mouse at 3 weeks post AdCre application, axial view. Tumour circled in red. ( b ) Corresponding CBCT scan of a KL mouse, ( a ) axial view (left panel), sagittal view (middle panel) and coronal view (right panel). Tumour circled in red. ( c ) Simulation of beam angles: red line represents 90° left lateral beam, white line represents 10° left dorsal beam. ( d ) Simulation of both involved fields (flanking blue lines) using a 5 × 5 mm 2 collimator. ( e ) Simulation of radiation dose distribution around the treatment volume. The prescribed dose was 8.5 Gy in one fraction. ( f ) Sagittal view of e (mouse head on the left). Rapid fall-off of the radiation dose beyond the prescribed isodose is visualized by colour wash. Full size image To confirm our targeting accuracy, we performed immunohistochemical analysis of γ-H2AX foci formation in a lung tumour from a K mouse 30 min after a single dose of radiation. In this experimental setup, the formation of γ-H2AX foci serves as a marker of RT-induced DNA double-strand breaks [19] . We used a square-shaped collimator (5 × 5 mm 2 ) that we knew a priori would not cover the complete tumour volume ( Supplementary Fig. 2 ). As expected, the square shape is accurately represented on the stained section and clearly distinguishes irradiated versus non-irradiated tissue. Tumour response of Kras -driven NSCLC to IGRT We next sought to determine whether the therapeutic effect of RT on tumour response kinetics is similar in mice and humans. As the translation of treatment doses used in humans to mice has not been well studied and is dependent on a number of complex biological factors (for example, differences in target volume size, species-specific radiation sensitivity), we decided to pick two different RT regimens that are commonly used for palliative treatment in humans [13] , [14] . Tumours were irradiated to a dose of 20 Gy in five fractions on five consecutive days (4 Gy × 5; Fig. 3a , top panel) or 17 Gy in two fractions of 8.5 Gy given on two consecutive days approximately 24 h apart (8.5 Gy × 2; Fig. 3a , bottom panel). After RT, tumour growth kinetics were evaluated every 2 weeks using non-invasive MRI. K mice treated with either 4 Gy × 5 ( Fig. 3b ) or 8.5 Gy × 2 ( Fig. 3c ) showed local tumour control (less than 30% volume reduction or less than 20% volume increase of the target lesion compared with baseline tumour volume) for 8 and 12 weeks, respectively, after RT. Comparison of treatment responses after these two RT regimens in tumours of K mice did not yield clear superiority of one regimen over the other. 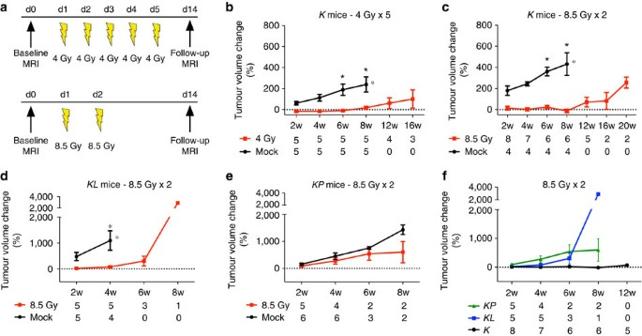Figure 3: Tumour response ofK, KLandKPmice after image-guided RT. (a) Schematic representation of two RT regimens used in this study. (b–f) Tumour growth kinetics inK(b,c),KL(d),KP(e) and all three genotypes (f, taken fromc–e) after RT. RT regimens are indicated on each graph. In all graphs, the tumour volume change compared with baseline is displayed for the indicated time points. Numbers below each time point indicate the number of mice evaluated at that time point per group. Data are represented as ±standard error (s.e.m.).Pvalues were calculated using a two-tailed Student’st-test. *P<0.05. °Indicates that these control groups had to be discontinued due to extensive tumour burden or death. w, weeks. Figure 3: Tumour response of K, KL and KP mice after image-guided RT. ( a ) Schematic representation of two RT regimens used in this study. ( b – f ) Tumour growth kinetics in K ( b , c ), KL ( d ), KP ( e ) and all three genotypes ( f , taken from c – e ) after RT. RT regimens are indicated on each graph. In all graphs, the tumour volume change compared with baseline is displayed for the indicated time points. Numbers below each time point indicate the number of mice evaluated at that time point per group. Data are represented as ±standard error (s.e.m.). P values were calculated using a two-tailed Student’s t -test. * P <0.05. °Indicates that these control groups had to be discontinued due to extensive tumour burden or death. w, weeks. Full size image We recently reported that the concomitant loss of tumour suppressors in Kras -driven murine NSCLC dramatically impacts the response to standard chemotherapy [4] . Given these genotype-dependent differences in treatment efficacy after systemic therapy, we analysed the tumour growth kinetics in KL and KP mice after 8.5 Gy × 2 ( Fig. 3d,e ). In comparison to K tumours, local tumour control in KL mice was decreased to 4 weeks, which was followed by substantial tumour progression ( Fig. 3d ). However, tumour response in KP mice appears to have distinct kinetics compared with K and KL tumours. Although RT treatment slows down KP tumour growth, no period of local tumour control could be observed ( Fig. 3e ). Whether lack of functional DNA damage response in these tumours accounts for these differences remains to be studied in further detail. Direct comparison of therapeutic efficacy in all three models ( Fig. 3f , taken from 3c,d,e) indicates prolonged local tumour control only in K mice. Although RT initially stabilizes KL tumour growth, the resultant rapid growth post-treatment suggests that these tumours have compensatory mechanisms to escape the effects of RT and that the addition of other anticancer agents will be needed to prolong local tumour control in this aggressive cancer. KP tumours appear to be the most intrinsically radioresistant as they have the least response to RT (8.5 Gy × 2). Whether dose escalation, modified delivery regimens or additional therapeutics can alter the treatment response should be addressed in future analyses. Radiobiologic effects of single fraction RT To determine whether a single fraction of RT was sufficient to induce DNA damage and subsequent cell death in vivo , we analysed tumours of K , KL and KP mice at several time points shortly after RT ( Fig. 4 ). In tumours of all three genotypes, we observed a profound increase of γ-H2AX foci formation within the first 30 min after a single dose of 8 Gy. Our data further show that γ-H2AX foci have returned back to baseline levels in all three genotypes by 12 h after the DNA-damaging insult ( Fig. 4a,b ). Although semi-quantitative evaluation of γ-H2AX foci across all K -driven tumours might suggest different DNA repair kinetics dependent on additional deletion of either p53 or Lkb1 , further detailed studies are required to address this question. Next, we analysed whether the proliferation rate was affected upon RT ( Fig. 4c ). Using Ki-67 staining as a surrogate for the proliferation rate, we observed considerable differences in the basal proliferation between the three genotypes ( K 36.8±4.26; KL 54.75±9.15 and KP 55.75±6.26 number of positive cells) and therefore normalized to untreated tumours to allow for meaningful comparisons between genotypes. A maximal decrease in protein expression was reached 8 h after 8 Gy IR. However, 24 h after the DNA-damaging insult, KL and KP tumours show similar Ki-67 expression levels compared with their untreated tumours, whereas K tumours seem to require more time to recover. Notably, KL tumours regain baseline proliferation rates as early as 12 h after RT, which could suggest for an elevated intrinsic radioresistance. We also performed cleaved caspase-3 staining as a marker for apoptotic cell death, and found increased expression 4–12 h after 8 Gy IR in all tumour types ( Fig. 4d ). We conclude that a single dose of 8 Gy is sufficient to induce double-strand breaks, temporarily decreases the proliferation rate and leads to apoptosis as one mechanism of cell death in our model. 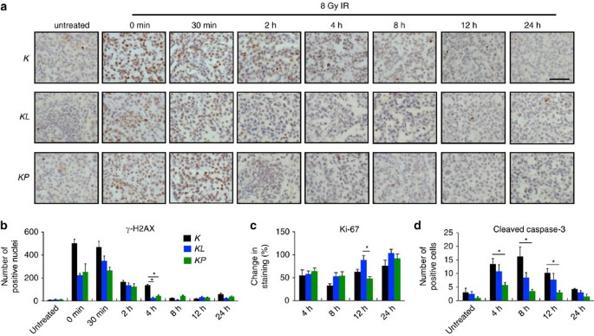Figure 4: Kinetics of double-strand break formation, proliferation rate and apoptotic signalling. (a)K, KLandKPmurine lung tumours were treated with a single dose of 8 Gy and the lungs were harvested at the indicated time points. Sections were stained for γ-H2AX foci. Scale bar, 50 μm. (b) Quantitative analysis of γ-H2AX-positive nuclei per field of view of the data presented ina. Quantification of Ki-67 (c) and cleaved caspase-3-positive cells (d) per microscopic field in mice of different genotypes of the same experiments. Data incare presented normalized to untreated tumours to allow for comparisons between genotypes given differences in the baseline proliferation. Data represent the average of 3–5 different fields ±standard error (s.e.m) from 1 to 3 different mice.Pvalues were calculated using a two-tailed Student’st-test. *P<0.05. Figure 4: Kinetics of double-strand break formation, proliferation rate and apoptotic signalling. ( a ) K, KL and KP murine lung tumours were treated with a single dose of 8 Gy and the lungs were harvested at the indicated time points. Sections were stained for γ-H2AX foci. Scale bar, 50 μm. ( b ) Quantitative analysis of γ-H2AX-positive nuclei per field of view of the data presented in a . Quantification of Ki-67 ( c ) and cleaved caspase-3-positive cells ( d ) per microscopic field in mice of different genotypes of the same experiments. Data in c are presented normalized to untreated tumours to allow for comparisons between genotypes given differences in the baseline proliferation. Data represent the average of 3–5 different fields ±standard error (s.e.m) from 1 to 3 different mice. P values were calculated using a two-tailed Student’s t -test. * P <0.05. Full size image The purpose of this study was to establish a preclinical platform for state-of-the-art delivery of IGRT. Highly predictive animal-based translational cancer research requires close analogy to the human setting. Optimal genetic and histopathological features of human NSCLC can be modelled by utilization of NSCLC-specific GEMMs. In this study, we used three highly relevant models of NSCLC: with Kras +/− Lkb1 or p53 (all commonly found to be mutated in human lung adenocarcinomas [20] ). In contrast to recent preclinical RT studies [8] , [9] , we developed a novel technique, which allows generation of Cre-mediated single lung tumours. The induction of a solitary tumour nodule closely recapitulates the human disease distribution at the time of diagnosis. Non-invasive imaging is necessary for timely tumour detection as definite clinical symptoms of disease burden are lacking. However, despite the technical challenges to apply this induction method and increased burden of screening for tumour-bearing mice, we believe that our induction method has further benefits in preclinical drug evaluation studies that are highly relevant to the treatment of localized disease. We expect that this model will provide a longer treatment evaluation period, as the right lung remains unaffected and compensates for impaired gas exchange in the left lung. Second, the increased survival of tumour-bearing mice also provides additional ‘tumour persistence time’, which could lead to additional genomic alterations and subsequent metastatic disease. In a subset of our intrathoracically induced mice, we found tumour lesions in the right lung. We are currently evaluating whether these were induced by ‘viral spillage’ through the respiratory airway system or whether these lesions are true metastases. Further differences of our study in contrast to others are the utilization of the small animal radiation research platform (SARRP) in conjunction with 3DCRT planning, which allows for precise irradiation with accurate delivery of dose to the tumour. As comprehensive studies on radiation-associated acute and long-term toxicities in various mouse tissues are missing, careful dose evaluation should be performed before any long-term treatment studies. During the course of our study, we did not observe any acute toxicities after 8.5 Gy × 2. Also, we did not observe signs of radiation pneumonitis, rib fractures or pleural effusions in K mice that had been on study for more than 12 weeks, although it is unclear whether an observation period of 12 weeks is sufficient for the development of these side effects. Future studies using this platform will be undertaken to address these critical clinical questions. We studied two dose fractionation schemes, 4 Gy × 5 and 8.5 Gy × 2, that are commonly employed clinically. Although the total radiation doses do not seem markedly different, variations in fraction size can have substantial biological impact. It is hypothesized that high doses per fraction above a threshold dose of 8–10 Gy lead to additional mechanisms of tumour control including antiangiogenic endothelial cell apoptosis [21] . Further studies of these mechanisms in our GEMM models may provide additional insights into the high efficacy of SBRT compared with conventional RT. For example, SBRT doses in human patients can produce control rates in excess of 90%. As we do not see this degree of efficacy in the doses utilized in this study, we will likely need to escalate the total dose to mirror the ablative (SBRT) treatments in human patients. However, the two schema used in this study provide an ideal platform to test the radiosensitization potential of various chemotherapeutic and targeted agents. Given our recent finding that additional loss of either Lkb1 or p53 has marked impact on the response to standard chemotherapy [4] , our present treatment data, proliferation and DNA damage repair kinetics further support the idea that underlying genetic alterations can serve as valuable biomarkers in stratifying patients with NSCLC for RT. Although further in-depth analyses are warranted to identify and validate the mechanisms leading to the observed genotype-dependent RT responses, the underlying biology might partially be explained on the basis of increased genomic instability in Lkb1- and p53- deficient lung tumours. In response to constant genotoxic stress, cells have evolved powerful DNA surveillance systems to maintain genomic integrity [22] . Defects in these checkpoint pathways fail to induce cell cycle arrest for proper DNA damage repair [23] . Thus, accumulation of unrepaired DNA lesions can promote malignant transformation. Our data suggest that K tumours have sufficient cell cycle checkpoints in place, as we observe stabilized disease burden for several weeks. However, the DNA-damaging assaults induced by IR might also affect checkpoint proteins and lead to re-growth of the tumour. Furthermore, our observations on tumour growth rates upon RT in KL and KP mice underscore the notion of dysfunctional cell cycle control mechanisms. Our novel RT platform provides all necessary requirements to further analyse and validate the underlying biological mechanisms of genotype-dependent RT responses in murine NSCLC. In summary, we provide evidence that it is feasible to induce single lung tumours in GEMMs of NSCLC. We further show that state-of-the-art IGRT can be precisely delivered to the murine lung without major impact on adjacent tissues. Comparison with clinical trials suggests that these GEMMs accurately mirror human responses. Therefore, we anticipate that validated GEMMs are useful in predicting outcome and interrogating mechanisms of therapeutic response and resistance. Viral vector production The Adeno-Cre virus was purchased from the Gene Transfer Vector Core Facility at the University of Iowa. The lentiviral vector Luc.Cre (Addgene, plasmid 20905) was packaged at Capital Biosciences, and concentrated to 1 × 10 7 IU ml −1 . Mice Mouse strains harbouring a conditional activating mutation (G12D) at the endogenous Kras locus, conditional Lkb1 knockout and conditional p53 knockout were described previously [11] . All experimental mice were maintained on a mixed genetic background (C57Bl/6, Balb-c, and S129). All in vivo experiments performed in this study were approved by the Animal Care and Use Committee of the Dana-Farber Cancer Institute. In vivo intrathoracic vector injection A maximum of 10 μl virus suspension was filled in insulin syringes (2.5 to 5 × 10 7 plaque-forming units of Adeno-Cre or 1 to 2 × 10 5 plaque-forming units of Lenti-Luc.Cre). Both virus preparations were diluted in DMEM and Adeno-Cre preparations were additionally precipitated with calcium chloride [16] . Male and female mice at the age of 5–10 weeks were anaesthetized with 1–3% isoflurane and positioned in right lateral decubitus for intrathoracic virus application into the left lung lobe. To assure aseptic skin puncture, the fur was clipped on the left chest and shoulder region using a cordless electric clipper. The shaved area was further cleaned with iodine and an alcohol pad. A 30-G needle attached to a 0.3 ml insulin syringe was used for the application of the virus. The needle was inserted at a 90° angle 1–2 mm caudal from the caudal angle of the scapula into the left lung at a depth of 3–5 mm (female mice are smaller and the injection depth needs to be adjusted). The caudal angle of the scapula served as an anatomic landmark to identify the injection site (roughly 4th or 5th intercostal space). Visualization of the caudal angle of the scapula was done by elevating the left forelimb. This manoeuvre was conducted without changing the position of the mouse. The insertion of the needle was performed on the cranial edge of the rip to prevent injury of subcostal nerves and vessels. After injection of the virus, the needle was quickly removed to minimize the risk of pneumothorax. In order to avoid ‘viral spillage’ to the contralateral lung, the mouse was positioned in left lateral decubitus until recovery from isoflurane anaesthesia. Every mouse was closely observed for abnormal breathing patterns suggestive for pneumothorax and other injection-related side effects (for example, bleeding from the injection site). Upon waking, the mice received one dose of buprenorphine (0.05–01 mg kg −1 ) subcutaneously for pain releave. There was a low morbidity associated with i th injections (<1%). Magnetic resonance imaging Mice were imaged on a 4.7-Tesla BioSpec 47/40 MRI scanner (Bruker BioSpin). Animals were anaesthetized with 1–3% isoflurane via a nose cone. A gradient echo flow compensated sequence using a repetition time of 372.5 ms, echo time of 7.0 ms and flip angle of 30° were used throughout the study. The slice thickness was 1 mm, and the number of slices was 17–20, which was sufficient to cover the entire lung. The acquisition matrix size was 256 × 128, the reconstructed matrix size was 256 × 256 and the field of view was 2.56 × 2.56 cm 2 . Motion artefacts were minimized by application of cardiac and respiratory gating to all MRI studies. All animals were scanned by using the described settings and parameters. Tumour volume quantification Tumour volume (mm 3 ) per animal was quantified by manual segmentation of the visible lung opacities present in each axial image sequence (a maximum of ten consecutive scans were evaluated per mouse) to calculate tumour volumes using 3D Slicer (version 3.6.3). All analysis was done in a blinded manner to treatment group and genotype. Currently, no standard response criteria exist to evaluate the effect of drug treatment on murine lung tumours. Contrary to human studies, which rely on uni- or bi-dimensional tumour measurements, we used tumour volume measurements to determine tumour treatment response as described previously [24] . Briefly, we applied the following criteria: (i) complete response=target lesion disappeared completely; (ii) partial response=at least 30% volume reduction of target lesion (compared with the baseline tumour volume); (iii) progressive disease=at least 20% volume increase of target lesion (compared with the baseline tumour volume) and (iv) stable disease=neither sufficient reduction or increase of tumour volume to qualify for partial response or progressive disease, respectively (compared with the baseline tumour volume). These are in keeping with RECIST response criteria used in human clinical studies. Bioluminescence imaging Bioluminescent imaging was performed on KLP mice induced with Lenti-Luc.Cre using a Xenogen IVIS Imaging System 100 from Caliper Life Sciences. Mice were intraperitoneal injected with 150 mg kg −1 D -luciferin (Caliper Life Science), anaesthetized with isoflurane and dorsal and left lateral images were then captured 5 min post luciferin injection. Small animal radiation research platform Mice were anaesthetized via isoflurane inhalation (1–3%) for the duration of each treatment. Before each treatment, CBCT using 65 kVp and 0.6 mA photons was performed on each mouse to visualize the tumour. All murine lung cancers were treated using a 1.2-cm circular collimator or a 5 × 5 mm 2 collimator using 220 kVp and 13 mA photons. Each fraction was applied in two equal en face fields (90° left lateral and 10° left dorsal). The SARRP Dose Planning System and 3D Slicer were used to precisely target murine lung cancers. Animals that served as untreated controls still underwent the stress of placement on the irradiation platform and also underwent CBCT imaging as often as the treated mice. The sample size N was determined using the estimated effect size from a dose defining pilot study and was calculated by an a priori analysis using G*Power (version 3.1.9.2). In all three genotypes, the baseline tumour volume before RT ranged between 50 and 200 mm 3 . Randomization was done in a blinded manner to treatment group and genotype. An ADCL-calibrated ion chamber was used to measure absolute dosimetry of the SARRP beam and Gafchromic film (EBT3) was used to measure percentage depth dose and profiles. The full procedure for commissioning a low-energy X-ray source can be found in the AAPM Task Group 61 Report [25] . Histology and immunohistochemistry Lungs were perfused with 10% formalin, stored in fixative overnight and embedded in paraffin. For further staining (haematoxylin/eosin and immunohistochemisty), sections of 5 μm were cut. Primary antibodies from Cell Signaling Technologies were used at the listed dilutions: phospho-Histone H2A.X (Ser139) (#20E3; 1:400), Cleaved Caspase-3 (Asp175) (#5A1E; 1:800). The Ki-67 antibody (16A8) was purchased from BioLegend and used at a dilution of 1:50. Positive cells were identified visually in each high-power field ( × 40 magnification). A total of 3–5 fields were observed per tumour. Statistical analysis Statistical analysis was performed with SPSS (version 22.0, SPSS Inc.). Differences between the groups were evaluated by one-way analysis of variance, Student-Newman-Keuls test and t -test where appropriate. Data are presented as mean±s.e.m., and P <0.05 was considered statistically significant. How to cite this article : Herter-Sprie, G. S. et al. Image-guided radiotherapy platform using single nodule conditional lung cancer mouse models. Nat. Commun. 5:5870 doi: 10.1038/ncomms6870 (2014).